Regional population collapse followed initial agriculture booms in mid-Holocene Europe Following its initial arrival in SE Europe 8,500 years ago agriculture spread throughout the continent, changing food production and consumption patterns and increasing population densities. Here we show that, in contrast to the steady population growth usually assumed, the introduction of agriculture into Europe was followed by a boom-and-bust pattern in the density of regional populations. We demonstrate that summed calibrated radiocarbon date distributions and simulation can be used to test the significance of these demographic booms and busts in the context of uncertainty in the radiocarbon date calibration curve and archaeological sampling. We report these results for Central and Northwest Europe between 8,000 and 4,000 cal. BP and investigate the relationship between these patterns and climate. However, we find no evidence to support a relationship. Our results thus suggest that the demographic patterns may have arisen from endogenous causes, although this remains speculative. Early farming economies spread into the Aegean from SW Asia by 8,500 years ago; by 8,000 years ago, they had spread north of the river Danube as far as present-day Hungary and Romania. At the same time, they spread along the north coast of the Mediterranean, reaching southern France around 7,800–7,700 years ago and Iberia shortly afterwards. From around 7,500 years ago there was a very rapid spread of farming practices across the loess plains of Central Europe, reaching the Paris Basin by c. 7,200–7,100 years ago. Subsequently, there was a standstill of c. 1,000 years before farming spread to Britain, Ireland and northern Europe c. 6,000 years ago [1] . There is increasing evidence from ancient DNA and other sources [2] , [3] that colonizing populations introduced farming over much of this area, although at the northern margins there may have been some adoption by indigenous hunter gatherers [4] , [5] , [6] . It has long been argued that the basis for expansion was new food production and consumption patterns [7] leading to increased population growth rates and higher population densities [8] . Ammerman and Cavalli-Sforza [9] showed that, to a first order of approximation, the overall rate of spread into Europe could be accounted for by the population ‘wave of advance’ model, first proposed by Fisher [10] , which assumes logistic population growth. Some years ago, Bocquet-Appel [11] demonstrated that the predicted demographic impact of farming could be detected by evidence for an increase in fertility, reflected in an elevated proportion of young individuals in European cemeteries at the time. Subsequently, this ‘Neolithic Demographic Transition’ has been shown to be a globally widespread phenomenon [11] , [12] , [13] . However, there have been few attempts to examine regional scale demography after the arrival of farming. It has been generally assumed that populations grew steadily, in line with long-term continental and global trends [14] . In this study, we examine summed calibrated date probability distributions (SCDPD) for 7,944 radiocarbon dates in 12 regions across western Europe as a demographic proxy and explore the relationship between human demography and climate [15] before, during and after the arrival of farming by cross-correlating changes in SCDPD-inferred population densities with seven climate proxies (see Methods , Fig. 1 ). In addition, we compare the spatial variability in recent climate between three adjacent sub-regions with contrasting demographic proxy patterns, and, on the assumption that prehistoric spatial climate variability would have been similar to that in the recent past, assess the extent to which this can account for the differences in the same sub-regions’ SCDPDs. 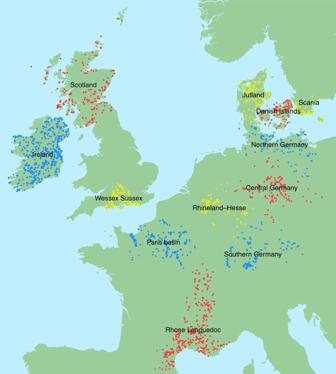Figure 1: Map of Central and North Western Europe. Points indicate archaeological site locations and colours delineate the sub-regions used to estimate demographic patterns. Figure 1: Map of Central and North Western Europe. Points indicate archaeological site locations and colours delineate the sub-regions used to estimate demographic patterns. Full size image Although age-at-death distributions give us an indication of changing fertility patterns at the continental scale [11] , [12] , and genetic data can be used to make inferences on population growth, decline and replacement, in principle neither approach can track local population density change with the spatiotemporal precision provided by radiocarbon dates from archaeological sites [16] . The basis for this demographic proxy is the assumption that there is a relationship between the number of dated archaeological sites falling within a given time interval in a given region (or their summed date probabilities) and population density [17] . Clearly, a variety of factors can potentially disturb this relationship. Sampling error could lead to misleading features in SCDPDs, particularly if sample sizes are small. In addition, spatiotemporal variation in site preservation and archaeological sampling biases, choice of samples to radiocarbon date, sample preparation contamination and laboratory protocols are all potential sources of systematic error [18] . Finally, the calibration curve itself demonstrates a non-monotonic relationship between 14 C production rates and time; therefore, the calibration process introduces date uncertainty [19] . Here we test the significance of fluctuations and autocorrelation in SCDPDs, and the cross-correlation between SCDPDs and climate proxy records, by using computer simulation of 14 C dates generated under a null model of exponential increase in the SCDPD through time as a result of population increase and better survival of the archaeological record towards the present. Our method accommodates numerous biases including sampling error, and potential spurious deviations and cross-correlations because of the calibration curve. We show that although populations did indeed grow rapidly in many areas with the onset of farming, the characteristic regional pattern is one of instability; of boom and bust. We find little evidence that, at the time scales considered, the variation in population levels through time is associated with climate, and that the very small variation in recent climate between three closely adjacent regions, if projected into the past, is not enough to explain the much larger inter-region variation in demography. We discuss other possible causes, and argue that whatever the cause, it is most likely endogenous and has to some extent affected demography in virtually all regions. Modelling population dynamics To a first order of approximation, we expect both preindustrial long-term human population growth [14] , and taphonomic processes [20] , to generate an exponential increase in dateable samples forward in time. For this reason we fitted an exponential generalized linear model (GLM; see Methods and Supplementary Table S1 ) with a quasi-Poisson distributed error to the SCDPD of all 13,658 dates in our database for western Europe, using a date range of 10,000–4,000 cal. BP ( Fig. 2 ) to provide an appropriate null model against which the hypothesis of booms and busts could be tested. 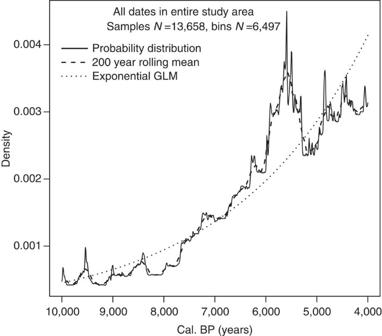Figure 2: SCDPD-inferred population density change 10,000–4,000 cal. BP using all radiocarbon dates in the western Europe database. The fitted null model of exponential population growth is used to calculate the statistical significance of regional (Fig. 3) and combined regional growth deviations (Fig. 4). Figure 2: SCDPD-inferred population density change 10,000–4,000 cal. BP using all radiocarbon dates in the western Europe database. The fitted null model of exponential population growth is used to calculate the statistical significance of regional ( Fig. 3 ) and combined regional growth deviations ( Fig. 4 ). Full size image We then tested the SCDPDs for the 12 regions in this specific study for departure from the null model ( Fig. 3 ). Ten of the 12—the exceptions are Central and north Germany—show evidence of a significant increase in population with the local appearance of farming, and then subsequently drop back to trend; populations in Scotland and Ireland drop significantly below trend. All regions except Central and North Germany show evidence of demographic fluctuations significant beyond expectation under our exponential null model, positive and/or negative and large in scale, over the course of the Neolithic (all data and demographic patterns are summarized in Table 1 ). For comparison, we also apply a bootstrap procedure to the SCDPDs as an alternative method of illustrating uncertainty in population density estimation ( Supplementary Fig. S1 ). It is important to note that strong support for these demographic patterns in Britain is found in independent evidence such as indicators of anthropogenic impact on forest cover from pollen diagrams [21] and the fluctuations in the number of directly dated cereal grains and hazel nut shells—indicators of subsistence type and intensity—from Neolithic and Bronze Age sites [22] . Similarly, independent support for the patterns shown in the Rhineland has been found [23] , [24] . 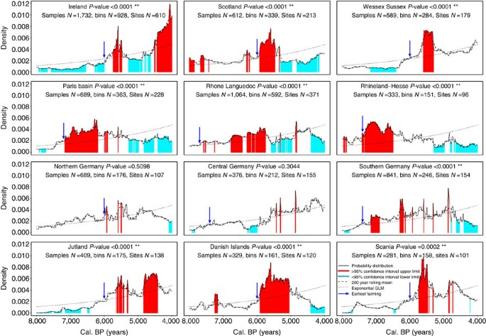Figure 3: SCDPD-inferred population density change 8,000–4,000 cal. BP for each sub-region. Statistically significant deviations from the null model (see Methods) are indicated in red and blue, and blue arrows indicate the first evidence for agriculture in each region. **P-values smaller thanP<0.0051, the 95% confidence level calculated using the Šidák correction (see Methods). Figure 3: SCDPD-inferred population density change 8,000–4,000 cal. BP for each sub-region. Statistically significant deviations from the null model (see Methods) are indicated in red and blue, and blue arrows indicate the first evidence for agriculture in each region. ** P -values smaller than P <0.0051, the 95% confidence level calculated using the Šidák correction (see Methods). Full size image Table 1 Regional summed radiocarbon date probability distributions analysis. Full size table We then tested the SCDPD of the 12 regions in our study combined for departure from the null model. There are significant positive deviations from the fitted exponential GLM, especially after 6,000 cal. BP. The later sixth and early-fifth millennia cal. BP, on the other hand, are characterized by densities significantly below the fitted GLM trend, before a return to trend at the end of the fifth millennium ( Fig. 4 ). 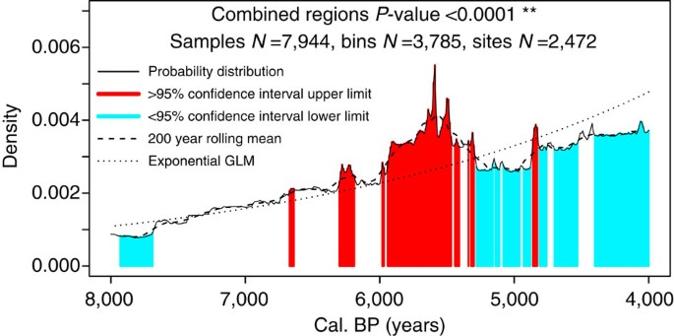Figure 4: SCDPD-inferred population density change 8,000–4,000 cal. BP for all regions combined. Statistically significant deviations from the null model of long-term growth (see Methods) are indicated in red and blue. Figure 4: SCDPD-inferred population density change 8,000–4,000 cal. BP for all regions combined. Statistically significant deviations from the null model of long-term growth (see Methods) are indicated in red and blue. Full size image Correlation with paleoclimate proxies There has been extensive discussion in the literature of the impact of climate on early farming populations in Europe [25] , [26] , [27] ; hence, the question arises whether the inferred demographic patterns correlate with paleoclimate. Cross-correlation analyses were performed using seven climate proxies (see Methods ). However, it is conceivable that any initially apparent correlations are not causal but rather reflect a relationship between climate and atmospheric 14 C levels or reservoir effects [28] . For example, δ 14 C residual values have been linked with lower levels of solar activity and the 11-year sunspot cycle [29] . Again, therefore, it was necessary to take into account the fluctuations in the calibration curve when comparing the climate proxy values with the SCDPD patterns (see Methods ). In most cases there is no correlation. In the small number of regions showing significant results at the 95% confidence level adjusted for the multiple testing of the regions the cross-correlations are similar at all lags, indicating only a very broad general trend of long-term correlation between climate and demographic proxies. The P -values are summarized in Table 2 and details of analyses for all regions and paleoclimate proxies can be found in Supplementary Fig. S2 . A comparison of recent spatial variation in temperature and precipitation with regional differences in demographic trajectories also produced negative results (see Methods , Supplementary Figs S3–S6 and Supplementary Tables S2 and S3 ). Table 2 Cross-correlation analysis of the SCDPD and seven paleoclimate proxies. Full size table Our analyses of SCDPDs have provided a new rigour in their treatment by addressing the problems caused by fluctuations in the calibration curve and by sampling variation in the available dates. They thus provide a basis for increased confidence in SCDPDs as valid demographic proxies. As noted above, in regions where independent evidence is available the validity of the SCDPD demographic proxy has been confirmed [30] . Moreover, most regions show more than one boom–bust pattern, contradicting suggestions that they are simply a result of a bias on the part of archaeologists towards trying to date the first appearance of farming in their region. Although the European population follows an approximately exponential long-term growth trend ( Fig. 2 ), considerable regional variation is evident. In virtually all the regions examined here, there are significant demographic fluctuations and in most there are indications at certain points of population decline of the order of the 30–60% estimated by historians for the much later Black Death [31] , although of course absolute population sizes during the Neolithic were much smaller than that during the Middle Ages. It is particularly important to note that the bust following the initial farming boom is found in two historically separate agricultural expansions, the first into Central Europe c. 7,500 years ago and the second into Northwest Europe 1,500 years later. It is possible that some of these regional declines represent out-migration to neighbouring areas rather than a real decline in numbers, for example, from the Paris Basin into Britain, but, in some cases, for example, Ireland, Scotland and Wessex, it is very clear that the rising and falling trends are roughly synchronous with one another—there is little indication of one going up as the others go down. On present evidence the decline in the initially raised population levels following the introduction of agriculture does not seem to be climate-related, but of course this still leaves open a variety of possible causes that remain to be explored in the future. One possibility is disease, as the reference to the Black Death above implies, although this would have to be occurring on multiple occasions at different times in different places, given the patterns shown. It is perhaps more likely that it arose from endogenous causes; for example, rapid population growth driven by farming to unsustainable levels, soil depletion or erosion arising from early farming practices, or simply the risk arising from relying on a small number of exploitable species [32] . However, these suggestions remain speculative and an autocorrelation analysis of the demographic data did not find evidence of a cyclical pattern, which would be one indicator of the operation of endogenous processes ( Supplementary Fig. S7 ). Regardless of the cause, collapsing Neolithic populations must have had a major impact on social, economic and cultural processes. Data A database of 13,658 radiocarbon dates and their contexts from the western half of temperate Europe in the period 10,000–3,500 cal. BP was collated from publications and public databases [33] , [34] , [35] , [36] , [37] , [38] , [39] , [40] , [41] . A number of distinct regions representing major areas of settlement during the Neolithic were selected: Ireland; Wessex and adjacent areas in southern England; Scotland; the Paris Basin and Normandy; the Rhone valley and adjacent areas; Jutland; the Danish Islands; Scania (southernmost Sweden); northern Germany; the lower Rhine-Hesse region; central Germany; and southern Germany, including the adjacent loess areas of eastern France. Similar to Collard et al . [17] , we took an inclusive approach to date selection from the available sources and excluded dates regarded as invalid by the laboratory, and those that were clearly incorrect in relation to the cultural context they claimed to be dating. All others were included on the grounds that the inclusion of imprecise dates and others that might not survive rigorous ‘chronometric hygiene’ tests would tend to obscure and smear any real fluctuations in population densities of interest to us, rather than accentuating them, and so have a conservative effect on hypothesis tests. Radiocarbon date calibration Radiocarbon dates and their associated errors were calibrated using scripts written in the ‘R’ programming language ( http://www.r-project.org/ ) and the IntCal09 calibration curve [42] . We used an arithmetical approach for reasons of speed, and because we were not considering stratigraphic information or using site-phase order as a Bayesian prior. Tests showed that our calibration method gave identical results to Oxcal [43] ( Supplementary Fig. S8 ). To correct for investigator bias and oversampling within sites, we grouped multiple dates from individual sites into non-overlapping phases, such that after ordering the dates at a site, the next date was only assigned to a new phase (or bin) if there were more than 200 14 C years between it and the previous date. Calibrated date probability distributions of samples from the same site phase were summed and normalized to unity, and the resulting distributions were then summed across site phases for a given region and again normalized to unity. Significance testing Some features of a SCDPD may appear to represent interesting demographic events [17] , or correlate with important archaeological, environmental or climate processes, when in fact they are a spurious consequence of sampling variation, and/or possibly arise from features of the calibration curve itself (see Introduction). For these reasons, we designed a number of statistical tests based on the generation of simulated SCDPDs under the null hypothesis of no departures from a long-term exponential trend. As calibrated time, rather than 14 C time, is expected to be colinear with calendar time, it was necessary to simulate random (under the null hypothesis) calendar dates and then uncalibrate, before randomly applying empirically derived errors and recalibrating. We focused on a calendar date range of 4,000–8,000 cal. BP, but to minimize ‘edge effects’ we included 14 C dates well outside that range. We fitted an exponential GLM with a quasi-Poisson distributed error to a SCDPD constructed from all 14 C dates from the entire study area, using the wider date range of 4,000–10,000 cal. BP ( Fig. 2 , Supplementary Table S1 ). Simulated SCDPDs (50,000) for each demographic region were generated by sampling n calendar dates from under the fitted GLM where n is the number of site phases in each region, and then converting to n 14 C dates by sampling from the calibration curve error at the corresponding calendar date. The simulated 14 C dates were rounded using a Monte Carlo method to give the same proportion of different date roundings as that used by 14 C laboratories, assigned errors by sampling with replacement from observed 14 C data errors, and then calibrated using the same procedure as for the observed data. Finally, the simulated calibrated date probability distributions were summed and normalized to unity. To test whether our observed SCDPDs contain features that deviate from expectation under the null hypothesis, we first calculated the local (10-year bins) mean of the 50,000 simulations, which we used to perform a local Z -score transformation on SCDPDs of both the observed data and each of the simulations. This was necessary to remove any underlying patterns caused by features of the calibration curve. Finally, local 95% confidence intervals (CIs) of the Z -scores and regions where the Z -scores exceeded the CIs were highlighted on the SCDPD. Although the above procedures identify features of the SCDPDs that occur outside the 95% CI expected under the null hypothesis, we would expect 5% (false positives) of the observed features to deviate from this (assuming no autocorrelation in date densities). It was therefore necessary to apply a single global statistic to test whether the sum of deviations across the whole period departed from expectation. The global statistic we chose was the sum of the Z -scores that exceeded the constructed CI. This global statistic is inherently conservative, as it treats a random distribution of positives in the same way as a low entropy cluster of positives, if their sums are equal. Indeed, it should be noted from the plots that points outside the 95% CI tend to be clustered (i.e. show low entropy). This global statistic calculated from the observed data was compared with the 95% CI in a one-tailed test using a distribution constructed from the same global statistic applied to the 50,000 simulations, which by definition were false positives. To account for the multiple testing of 12 independent regions, a more rigorous CI was applied using the Šidák correction, which approximates to 99.51% CI ( Table 1 ). Climate correlation In addition to identifying significant features in the SCDPDs, we were also interested in testing for correlations between this demographic proxy and seven climate proxies (GICC05 (ref. 44 ), Crag Cave δ 18 O [45] , the Abisko valley chironomid-based temperature record from northern Sweden [46] , the winter precipitation record from the Aspvatnet glacial lake in northern Norway [47] and two separate North Atlantic sea surface temperature proxies, RAPiD-12-1K [48] and GIK 23258-2 (ref. 49 )). To account for uncertainty in the calibration curve, both simulated and real residuals were cross-correlated with the climate proxies, all interpolated to the 10-year resolution of the demography for consistency, and 95% CIs were calculated from simulated correlation coefficients. To take into account the possibility of false positives, each region’s cross-correlation distribution was then tested for significance in a one-tailed test that compared a single global statistic (the absolute value of the largest correlation coefficient) from each simulation with the real data, by considering whether this statistic falls outside the 95% CI of the simulated distribution of the same statistic for that single region. To account for the multiple tests of 12 data sets, we again applied the Šidák correction ( Table 2 and Supplementary Fig. S2 ). To further investigate the relationship between population and climate, we also compared historic (1 October 1972–14 January 1996) spatial variation in temperature and precipitation from weather station instrumental data of three closely adjacent regions at the same latitude—Jutland, Scania and the Danish Islands ( Supplementary Fig. S3 , Supplementary Table S2 ). Their historic temperature and precipitation patterns are all highly correlated ( Supplementary Figs S4–S6 , Supplementary Table S3 ), suggesting that their paleoclimates would also have been extremely similar to each other, and although the inferred demographic patterns of the first two regions have similar trajectories, the third is very different ( Fig. 3 ), indicating that climatic variation cannot account for the differences between them. In the light of the negative results of the climate analysis, an autocorrelation analysis of the demographic series was carried out on each region’s residuals to see whether they provided evidence of endogenous cyclicity ( Supplementary Fig. S7 ). This analysis was performed to explore lags between 0 and 1,000 years by using a ‘sliding window’ of 3,000 years to avoid imputing data outside the window of overlap. CIs were generated by repeating this process on each of the 50,000 simulations and estimating the local 95% CI. No evidence of cyclicity (typically characterized by at least one peak of positive correlation preceded by a peak of negative correlation at half the wavelength) was observed. In some regions, a positive correlation outside 95% CI was observed, suggesting a broad long-term autocorrelation because of a long-term increase or decrease. This result is in agreement with visual inspection of the SCDPDs. Bootstrap analysis As an alternative method of illustrating uncertainty in estimated population density because of sampling error in SCDPDs, we applied a bootstrap procedure ( Supplementary Fig. S1 ). Within each region, uncalibrated dates were repeatedly sampled with replacement, calibrated and plotted to construct a running CI through calendar time. In most cases, there appears to be a marked demographic expansion after the first evidence of agriculture, followed by population declines. How to cite this article: Shennan, S. et al . Regional population collapse followed initial agriculture booms in mid-Holocene Europe. Nat. Commun. 4:2486 doi: 10.1038/ncomms3486 (2013).